Mercury nano-trap for effective and efficient removal of mercury(II) from aqueous solution Highly effective and highly efficient decontamination of mercury from aqueous media remains a serious task for public health and ecosystem protection. Here we report that this task can be addressed by creating a mercury ‘nano-trap’ as illustrated by functionalizing a high surface area and robust porous organic polymer with a high density of strong mercury chelating groups. The resultant porous organic polymer-based mercury ‘nano-trap’ exhibits a record-high saturation mercury uptake capacity of over 1,000 mg g −1 , and can effectively reduce the mercury(II) concentration from 10 p.p.m. to the extremely low level of smaller than 0.4 p.p.b. well below the acceptable limits in drinking water standards (2 p.p.b. ), and can also efficiently remove >99.9% mercury(II) within a few minutes. Our work therefore presents a new benchmark for mercury adsorbent materials and provides a new perspective for removing mercury(II) and also other heavy metal ions from contaminated water for environmental remediation. Mercury (Hg) pollution, which can cause birth defects, brain damage, and disease in humans and other species, has long been a threat to public health and environment [1] . The release of mercury into environments is mainly through discharge from industry products/byproducts and processes, such as chemicals, electronic materials, batteries and fossil fuel combustion [2] . A global agreement has recently been reached aiming at reducing mercury’s threat, which spurs the research needed to remove and recover mercury ions from industry waste water [3] . An upper limit of 2 p.p.b. for mercury in drinking water has been mandated by the United States Environmental Protection Agency (EPA) [4] , and even much lower limits have been strictly regulated for the discharge of mercury into aquatic systems to protect ecosystems [5] . Among various technologies developed over the years for mercury removal, adsorption holds great promise due to the simplicity and relatively low-cost of adsorption technology as well as the effectiveness of adsorption method to purify water [6] . A variety of adsorbents have been developed and tested for removing Hg(II) from contaminated waters. Conventional adsorbents such as activated carbons [7] , zeolites [8] and clays [9] generally have low capacity and weak binding affinity for mercury. Thiol/thio-functionalized adsorbents, including clays [10] , resins [11] , mesoporous silica [12] , [13] , [14] , [15] , [16] , activated carbons [17] , mesorporous carbons [18] and chalcogenides [19] , [20] , are considered very effective sorbents for Hg(II) removal from aqueous solutions due to the soft–soft interaction [21] . Recently, metal-organic frameworks (MOFs) [22] , [23] , [24] , [25] , [26] , [27] , [28] have been explored as a new type of adsorbents for mercury removal [29] , [30] , [31] , [32] , [33] , [34] due to their high surface areas, but they usually suffer from instability in water [29] , [30] or aqueous solutions with a wide pH range [34] and possess low adsorption capacity and weak affinity for Hg(II). Until now, existing adsorbent materials still face sorts of challenges such as the low surface area and improper distribution of thio/thiol groups thereby low capacity and moderate affinity for Hg(II), leaching of sulfur element and poor stability in a wide pH range, which have largely limited their effectiveness and efficiency for the removal of Hg(II) from aqueous solutions. The weaknesses and handicaps associated with existing adsorbents necessitate the development of new types of materials for highly effective and highly efficient removal of Hg(II) from aqueous solutions. To tackle the aforementioned challenges, in this contribution we illustrate a new approach by creating mercury ‘nano-trap’ ( Fig. 1 ) that features high surface area with densely populated yet highly accessible Hg(II) binding sites thereby affording high Hg(II) adsorption capacity; strong Hg(II) chelating groups that are well dispersed throughout the single-walled pore surface thus rendering high affinity for Hg(II) and efficient utilization of Hg(II) binding sites; large yet tunable pore size to enable fast yet controllable kinetics of Hg(II) adsorption; Hg(II) chelating groups that are covalently anchored to the backbone thus avoiding the leaching of binding sites; exceptional water/chemical stability facilitating regeneration/recyclability. Such mercury ‘nano-trap’ can be targeted by grafting desired Hg(II) chelating groups to the highly robust porous organic polymers (POPs) [35] , [36] , [37] , [38] , [39] , [40] , [41] , [42] , [43] , [44] that exhibit high surface areas, tunable pore sizes and high water/chemical stabilities, via stepwise post-synthetic modification [45] of the phenyl rings of their structural components using various established organic reactions. Herein we demonstrate such a POP-based mercury ‘nano-trap’ that exhibits an exceptional mercury saturation uptake capacity of over 1,000 mg g −1 and can effectively reduce Hg(II) concentration from 10 p.p.m. to the extremely low level of smaller than 0.4 p.p.b. and can efficiently remove >99.9% mercury within a few minutes, outperforming the performances of existing mercury removal adsorbents. Moreover, the POP-based mercury ‘nano-trap’ is highly effective for mercury removal over a very broad pH range and can be readily regenerated and recycled without significant loss of mercury adsorption capacity. 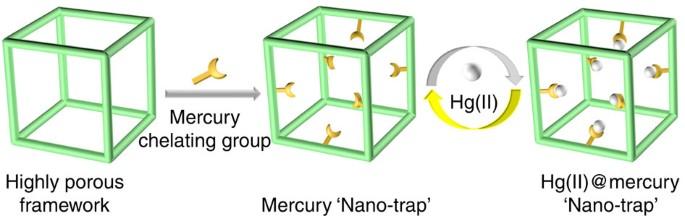Figure 1: ‘Nano-trap’ for Hg(II) removal. Illustration of creating mercury ‘nano-trap’ for Hg(II) removal from water. Figure 1: ‘Nano-trap’ for Hg(II) removal. Illustration of creating mercury ‘nano-trap’ for Hg(II) removal from water. Full size image Synthesis and characterization The POP-based mercury ‘nano-trap’ was afforded by functionalizing PAF-1 (ref. 46 ) (also known as PPN-6 (ref. 38 )), an amorphous POP ( Supplementary Fig. 1 ) that exhibits very high surface area and exceptional water/chemical stability, with thiol groups that are well-known to bind Hg(II) strongly. The thiol-functionalized PAF-1 (PAF-1-SH) was prepared by chloromethylation of PAF-1 followed by the treatment with NaHS ( Supplementary Figs 2 and 3 ). The successful grafting of thiol group onto PAF-1 was confirmed by Fourier transform infrared spectroscopy (FT-IR), X-ray photoelectron spectroscopy (XPS) and solid-state 13 C NMR studies. The FT-IR spectra of the dehydrated PAF-1-SH show the aliphatic C-H stretching bands at 2,959 cm −1 and 2,928 cm −1 as well as the characteristic band [47] of S-H at 2,576 cm −1 compared with the pristine PAF-1 ( Supplementary Fig. 4 ). XPS spectra of PAF-1-SH indicate the appearance of sulfur signal at a binding energy of 163.8 eV ( Supplementary Fig. 5 ), which is consistent with the S(2p) of the thiol group [48] . Solid-state 13 C NMR studies identify the chemical shifts at 23.0 and 28.9 p.p.m. for the carbon of –CH 2 group ( Supplementary Fig. 6 ), suggesting the successful attachment of –CH 2 SH groups to the phenyl rings in PAF-1. Elemental analysis reveals a sulfur content of 17.6 wt.% corresponding to 5.5 mmol g −1 –SH groups in PAF-1-SH, which indicates 57% of the phenyl rings are grafted with one –CH 2 SH group each. Nitrogen gas sorption isotherms collected at 77 K indicate that the grafting of thiol groups leads to a decrease in the Brunauer–Emmett–Teller (BET) surface area from 4,715 m 2 g −1 for PAF-1 to 3,274 m 2 g −1 for PAF-1-SH and a small reduction in pore size by about 3 Å ( Fig. 2b ). It is worth noting that the surface area of PAF-1-SH is significantly higher than any other thiol-modified porous materials, which usually exhibit moderate surface areas of 500~2,000 m 2 g −1 (refs 7 , 8 , 9 , 10 , 11 , 12 , 13 , 14 , 15 , 16 , 17 , 18 , 19 , 20 , 29 , 31 , 32 , 33 ). In addition, the sulfur content in PAF-1-SH is also remarkably higher compared with thiol group functionalized mesoporous silica MCM-41 (MCM-41-SH) (17.6 wt.% in PAF-1-SH versus 4.99 wt.% in MCM-41-SH). The high surface area and densely populated thiol groups prompt us to evaluate PAF-1-SH as mercury ‘nano-trap’ for Hg(II) removal from aqueous solutions. 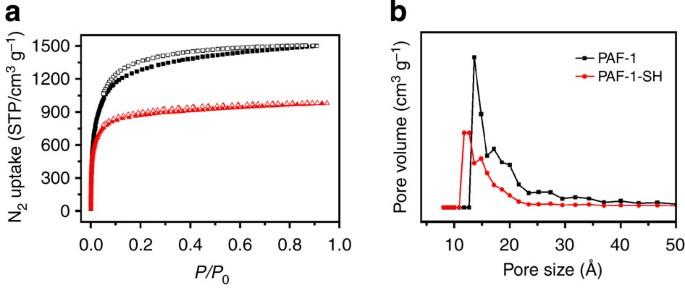Figure 2: N2sorption isotherms and pore size distributions. (a) N2sorption isotherms of PAF-1 (black) and PAF-1-SH (red). (b) Pore size distributions of PAF-1 (black) and PAF-1-SH (red). Figure 2: N 2 sorption isotherms and pore size distributions. ( a ) N 2 sorption isotherms of PAF-1 (black) and PAF-1-SH (red). ( b ) Pore size distributions of PAF-1 (black) and PAF-1-SH (red). Full size image Hg(II) sorption studies To evaluate the effectiveness of PAF-1-SH as mercury ‘nano-trap’ for removing Hg(II) from water, an as-made PAF-1-SH sample was placed in a dilute aqueous solution (pH of 6.8) of Hg(NO 3 ) 2 with Hg(II) concentration of 10 p.p.m. The adsorbed Hg(II) was observed by Energy-dispersive X-ray spectroscopy (EDS) spectra and sulfur from the thio group was also detected by EDS ( Supplementary Fig. 7 ). As shown in Fig. 3a , PAF-1-SH can rapidly capture Hg(II) ions; and after ~6 h the residual Hg(II) concentration in the solution was smaller than 0.4 p.p.b., that is, almost 99.997% of the mercury was removed by PAF-1-SH under such condition. It is noteworthy that the residual Hg(II) concentration in the solution treated with PAF-1-SH is 28 times lower than that (0.01 p.p.m.) in the solution treated with the MOF of Zr-DMBD [34] , and is also lower than that in the solution treated with thiol group functionalized FMMS (0.8 p.p.b.) (ref. 12 ) or Chalcogel-1 (0.04 p.p.m.) (ref. 19 ). These results therefore highlight the superior effectiveness of PAF-1-SH for removing Hg(II) from aqueous solutions compared with some benchmark sorbents. Indeed a single treatment of highly contaminated water with PAF-1-SH can effectively reduce the mercury concentration to well below U.S. Environmental Protection Agency elemental limits for hazardous wastes and even the acceptable limits in drinking water standards ( ≪ 2 p.p.b.) [4] . We reasoned that the high effectiveness of PAF-1-SH for mercury removal from aqueous solutions should be attributable to its high affinity for Hg(II) as a result of the highly accessible thiol groups that are densely populated throughout the inner surface of PAF-1-SH. 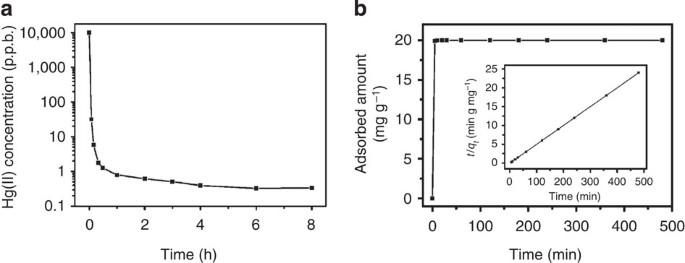Figure 3: Kinetics investigation of PAF-1-SH. (a) Hg(II) sorption kinetics of PAF-1-SH under the Hg(II) initial concentration of 10 p.p.m. (b) Adsorption curve of Hg(II) versus contact time in aqueous solution using PAF-1-SH. Inset shows the pseudo-second-order kinetic plot for the adsorption (Hg(II) concentration: 10 p.p.m.). Figure 3: Kinetics investigation of PAF-1-SH. ( a ) Hg(II) sorption kinetics of PAF-1-SH under the Hg(II) initial concentration of 10 p.p.m. ( b ) Adsorption curve of Hg(II) versus contact time in aqueous solution using PAF-1-SH. Inset shows the pseudo-second-order kinetic plot for the adsorption (Hg(II) concentration: 10 p.p.m.). Full size image One measure of a sorbent’s affinity for a target metal ion is the distribution coefficient ( K d ) measurement [49] . The K d is defined as: where C i is the initial metal ion concentration, C f is the final equilibrium metal ion concentration, V is the volume of the treated solution (ml) and m is the mass of sorbent used (g). The K d represents an important aspect of any sorbent’s performance metrics of metal ion adsorption, and K d values of 1.0 × 10 5 ml g −1 are usually considered excellent [18] . The K d of PAF-1-SH for Hg(II) has been measured to be exceptional with a value of 5.76 × 10 7 ml g −1 . This value is among the highest for sorbent materials for Hg(II) adsorption reported thus far, and exceeds that reported for a series of benchmark materials, for example, commercial resins (10 4 ~5.10 × 10 5 ml g −1 ) [50] , FMMS (3.4 × 10 5 ~1.68 × 10 7 ml g −1 ) [12] , [13] thiopyrene-functionalized mesoporous carbon (6.82 × 10 5 ml g −1 ) [18] , LHMS-1 (6.4 × 10 6 ml g −1 ) [50] , Chalcogel-1 (1.61 × 10 7 ml g −1 ) [19] and the MOF of Zr-DMBD (9.99 × 10 5 ml g −1 ) [34] . The efficiency of PAF-1-SH as mercury ‘nano-trap’ for removing Hg(II) from aqueous solutions has been examined by investigating the mercury adsorption kinetics of PAF-1-SH (25.0 mg) in 10 p.p.m. solution (pH of 6.8) of Hg(NO 3 ) 2 (50.0 ml). As shown in Fig. 3b , extremely fast kinetics are observed for PAF-1-SH, which can attain 99.9% of the adsorption capacity at equilibrium within 7 min and is able to reduce a heavily contaminated water with the Hg(II) concentration of 10 p.p.m. to the acceptable limit of 2 p.p.b. for drinking water within ≪ 20 min of PAF-1-SH/water contact ( Fig. 3a ). Considering the great reliability to represent the kinetics for the adsorption of heavy metal ions from aqueous solutions onto adsorbents [51] , the experimental data were fitted with the pseudo-second-order kinetic model using the following equation: where k 2 (g mg −1 min −1 ) is the rate constant of pseudo-second-order adsorption, q t (mg g −1 ) is the amount of Hg(II) adsorbed at time t (min), and q e (mg g −1 ) is the amount of Hg(II) adsorbed at equilibrium. An extremely high correlation coefficient (>0.9999) was obtained ( Fig. 3b ), and the value of the adsorption rate constant k 2 was determined to be 8.13 g mg −1 min −1 . This value is one or two orders of magnitude higher than other adsorbent materials for Hg(II) adsorption under similar conditions [32] , [52] , [53] , [54] , and such extraordinarily fast kinetics observed for PAF-1-SH can be ascribed to its large pore size adequately to facilitate the diffusion of Hg(II) ions and its high surface area densely populated with thiol groups. To assess the mercury uptake capacity of PAF-1-SH, which is also an important aspect of sorbent’s performance metrics, adsorption isotherm for Hg(II) removal from water (pH of 6.8) was collected ( Fig. 4 ). The equilibrium adsorption isotherm data were fitted with Langmuir model [34] , [52] yielding a high correlation coefficient (>0.9984) ( Fig. 4 inset). Remarkably, the maximum mercury adsorption capacity of PAF-1-SH was calculated to be 1,014 mg g −1 (~5.1 mmol g −1 ). This corresponds to the capture of 0.927 Hg(II) ion per thiol group in PAF-1-SH, suggesting the accessibility of almost all thiol groups in PAF-1-SH for Hg(II) ions. To the best of our knowledge, the maximum mercury uptake capacity of PAF-1-SH is the highest among adsorbent materials reported thus far for mercury adsorption, and is significantly higher than that of some benchmark thiol/thio-functionalized porous materials, for example, thiol-monolayer-functionalized mesoporous silica (505~600 mg g −1 ) [12] , [13] , thiopyrene-featured porous carbon (518 mg g −1 ) [18] Chalcogel-1 (645 mg g −1 ) [19] MOF Zr-DMBD (197 mg g −1 ) [34] . Such an outstanding saturation mercury uptake capacity can be attributed to the high surface area together with a large number of highly accessible thiol groups that are well dispersed throughout the inner surface of PAF-1-SH. 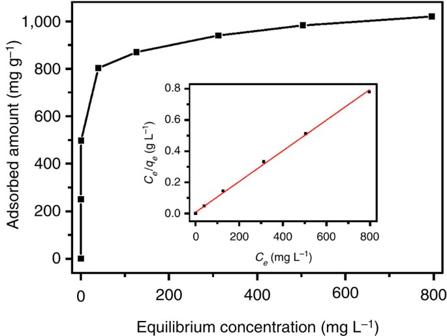Figure 4: Hg(II) adsorption isotherm for PAF-1-SH. Inset shows the linear regression by fitting the equilibrium adsorption data with Langmuir adsorption model. Figure 4: Hg(II) adsorption isotherm for PAF-1-SH. Inset shows the linear regression by fitting the equilibrium adsorption data with Langmuir adsorption model. Full size image The ability to withstand a variety of harsh chemical conditions (for example, extreme pH) and still effectively adsorb Hg(II) is highly desirable for a material in practical application of decontaminating Hg(II) from aqueous media [18] . The chemical/water stability of PAF-1-SH was verified by virtually no surface area drop after PAF-1-SH sample was treated successively with 2.0 M NaOH, 2.0 M HCl and boiling water, as revealed by N 2 sorption isotherms collected at 77 K ( Supplementary Fig. 8 ). This represents an advantage of PAF-1-SH for mercury removal across a wide range of pH, particularly when compared with silica and MOFs based adsorbents [12] , [13] , [14] , [15] , [16] , [29] , [30] , [31] , [32] , [33] , [34] , which usually suffer from the loss of porosity under such harsh conditions. Mercury adsorption experiments under acid and basic conditions revealed that PAF-1-SH also exhibits high affinities for Hg(II) with K d values of 6.66 × 10 7 ml g −1 at pH 1.0 and 2.49 × 10 7 ml g −1 at pH 12.8, which render excellent capability of reducing Hg(II) concentrations from 10 p.p.m. to ≪ 0.3 p.p.b. at pH 1.0 and ≪ 0.8 p.p.b. at pH 12.8 ( Supplementary Fig. 9 ). These results highlight the effectiveness of PAF-1-SH as mercury ‘nano-trap’ for removing Hg(II) from aqueous media over a broad range of pH values. The mercury-loaded PAF-1-SH can be regenerated by washing with a concentrated HCl (12.0 M) solution, which results in 100% removal of the loaded mercury. The regenerated PAF-1-SH retained >90% of the original loading capacity even after several regeneration and reuse cycles ( Supplementary Fig. 10 ). We reasoned that such excellent recyclability with negligible loss of mercury adsorption capacity observed for PAF-1-SH should be attributed to the well dispersive distribution of thiol groups throughout its highly porous framework structure thus minimizing the formation of the weaker binding S−S units as a result from the oxidation –SH groups. This is supported by the absence of S−S stretching bands (500–540 cm −1 ) [47] in the FT-IR spectra of regenerated PAF-1-SH ( Supplementary Fig. 11 ). The selectivity tests were also performed on PAF-1-SH in a Hg(II) solution containing Pb(II), Cd(II), As(III), Ca(II), Mg(II), Zn(II) and Na(I) ions ( Table 1 ). PAF-1-SH not only can effectively adsorb Hg(II), but also can largely remove other highly toxic heavy metal ions of Pb(II) and Cd(II). In contrast, other background metal ions such as Ca(II), Zn(II), Mg(II) and Na(I) do not quite bind to PAF-1-SH, and PAF-1-SH can remain effective in the presence of high concentrations of these ions. Similar results ( Table 2 ) were also obtained in the breakthrough experiments of passing the mixture solution of these ions through a column packed with PAF-1-SH. Similar to FMMS [12] , the high selectivity of Hg(II) and other heavy metal ions of Pb(II) and Cd(II) against the background metal ions of Ca(II), Zn(II), Mg(II) and Na(I) observed for PAF-1-SH should stem from the strong soft–soft interactions between Hg(II)/Pb(II)/Cd(II) ions and the thiol groups within PAF-1-SH. PAF-1-SH also exhibits low binding ability for As(III), and this should be due to that As(III) is a non-metal ion and exists in the form of AsO 2 − in aqueous solution, which can hardly interact with the thiol group strongly. Table 1 Concentrations of metal ions before and after the treatment of PAF-1-SH. Full size table Table 2 Concentrations of metal ions before and after the breakthrough experiments of PAF-1-SH. Full size table Investigation of Hg(II) binding interactions The outstanding performances of PAF-1-SH as mercury ‘nano-trap’ can be traceable to the strong binding interactions between Hg(II) and thiol group in PAF-1-SH, which have been elucidated by FT-IR, NMR and photoluminescence (PL) studies. As shown in Fig. 5a , IR spectra reveal a large shift of S−H stretch mode from 2,576 cm −1 in PAF-1-SH to 2,380 cm −1 in the Hg(II)-loaded PAF-1-SH, indicating the formation of strong binding interactions between Hg(II) and thio group. The formation of strong chemical bonding between the mercury and thiol group is also suggested by solid state 13 C NMR spectrum for Hg(II)-loaded PAF-1-SH ( Fig. 5b ), which indicates a large shift of 6 p.p.m. for the peak corresponding to the carbon (C6/C6′) attached to the thiol group. The strong binding interactions between Hg(II) and thiol group in PAF-1-SH are further evidenced by PL studies, which reveal that the PL intensity of PAF-1-SH host framework is greatly impacted by the Hg(II) uptake. As shown in Fig. 5c , the as-made sample features a broad emission centred around 420 nm, and the PL intensity is largely suppressed on the loading of Hg(II), being ≪ 1/3 of the intensity for the host PAF-1-SH. 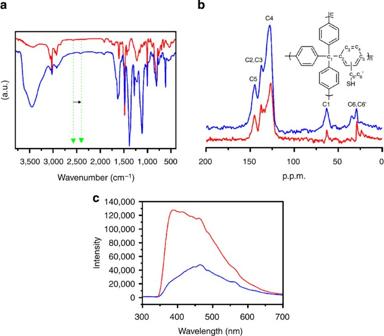Figure 5: Spectroscopic analysis of Hg(II) binding interactions. (a) FT-IR spectra of PAF-1-SH (red) and Hg(II)-loaded PAF-1-SH (blue). (b) Solid state13C NMR of PAF-1-SH (red) and Hg(II)-loaded PAF-1-SH (blue). (c) The PL spectra of PAF-1-SH (red) and Hg(II)-loaded PAF-1-SH (blue). Figure 5: Spectroscopic analysis of Hg(II) binding interactions. ( a ) FT-IR spectra of PAF-1-SH (red) and Hg(II)-loaded PAF-1-SH (blue). ( b ) Solid state 13 C NMR of PAF-1-SH (red) and Hg(II)-loaded PAF-1-SH (blue). ( c ) The PL spectra of PAF-1-SH (red) and Hg(II)-loaded PAF-1-SH (blue). Full size image To evaluate a material for mercury removal from aqueous solutions, the distribution coefficient ( K d ) and saturation uptake capacity have been deemed as two most important criteria, and high values for both of them are needed to achieve high effectiveness and high efficiency for mercury removal. Exceptional distribution coefficient for Hg(II) and extraordinary mercury saturation uptake capacity have both been demonstrated in the POP-based mercury ‘nano-trap’ of PAF-1-SH as reported herein, which sets a new benchmark for mercury adsorbent materials ( Fig. 6 ). The issues of structure stability under harsh chemical conditions, decreasing mercury affinity over a broad range of pH and loss of mercury uptake capacity on regeneration represent some barriers for most mercury adsorbent materials to be applied in practical application of decontaminating Hg(II) from aqueous media; these issues have also been well addressed in the POP-based mercury ‘nano-trap’ of PAF-1-SH. A high selectivity of Hg(II) against a series of trace metal ions (for example, Ca(II), Zn(II), Mg(II), Na(I)) represents another necessary consideration for mercury removal from aqueous solutions in reality, and this has been well demonstrated by the POP-based mercury ‘nano-trap’ of PAF-1-SH as well. The decent thermal stability up to 270 °C ( Supplementary Fig. 12 ) for PAF-1-SH suggests its capability for mercury vapour sorption, which is related to the industrial processes of flue gas detoxification [55] ; this aspect of work will be conducted in the near future. Albeit the high cost of PAF-1 would be a concern for the practical utilization of PAF-1-SH for mercury removal, the mercury ‘nano-traps’ can be readily achieved in other POPs [35] that are constructed from various organic building blocks derived from a variety of resources through economical reaction processes, thus paving a way to develop ‘nano-traps’ as a new platform for mercury removal. 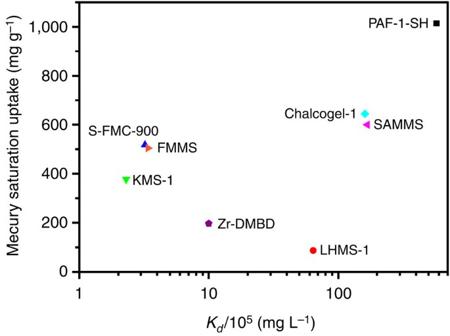Figure 6: Hg(II) saturation uptake. Comparision of Hg(II) saturation uptake amount andKdvalue for PAF-1-SH with other benchmark porous materials, KMS-1 (ref.56); LHMS-1 (ref.50); FMMS (ref.12); Chalcogel-1 (ref.19); S-FMC-900 (ref.18); Zr-DMBD (ref.34); SAMMS (ref.57); [a]:Kdvalue referred herein was measured based on the same initial concentration with others). Figure 6: Hg(II) saturation uptake. Comparision of Hg(II) saturation uptake amount and K d value for PAF-1-SH with other benchmark porous materials, KMS-1 (ref. 56 ); LHMS-1 (ref. 50 ); FMMS (ref. 12 ); Chalcogel-1 (ref. 19 ); S-FMC-900 (ref. 18 ); Zr-DMBD (ref. 34 ); SAMMS (ref. 57 ); [a]: K d value referred herein was measured based on the same initial concentration with others). Full size image In conclusion, we have demonstrated the creation of mercury ‘nano-trap’ for highly effective and highly efficient removal of Hg(II) from aqueous solutions as exemplified in the context of thiol-functionalized POP of PAF-1, PAF-1-SH. PAF-1-SH exhibits very high affinity for Hg(II) with an exceptional distribution coefficient value of 5.76 × 10 7 ml g −1 , extremely fast kinetics for Hg(II) adsorption with an extraordinary pseudo-second-order adsorption rate constant of 8.13 g mg −1 min −1 , and record-high saturation mercury uptake capacity of 1,014 mg g −1 . As mercury ‘nano-trap’, PAF-1-SH not only can effectively reduce Hg(II) concentration from 10 p.p.m. to the extremely low level of ≪ 0.4 p.p.b. well below the acceptable limits in drinking water standards ( ≪ 2 p.p.b.) and efficiently remove >99.9% mercury(II) within a few minutes, but also can retain high effectiveness for mercury removal over a very broad pH range and maintain high mercury adsorption capacity on regeneration and reuse; in addition, it can remain effective in the presence of high concentrations of background metal ions of Ca(II), Zn(II), Mg(II) and Na(I). Our approach of creating mercury ‘nano-traps’ based on highly porous and highly robust POPs thereby provides a new perspective for decontaminating Hg(II) from aqueous media. Moreover, the ‘nano-traps’ advanced herein can also be readily applied to capturing other heavy metal ions from contaminated water for environmental remediation as preliminarily demonstrated here, and the details of this aspect of work are currently under continuation in our laboratory. Materials and measurements Commercially available reagents were purchased in high purity and used without further purification. Powder X-ray diffraction (PXRD) data were collected on a Bruker AXS D8 Advance A25 Powder X-ray Diffractometer. N 2 gas sorption experiments were carried out on a Micrometrics ASAP2020 volumetric gas sorption instrument. Elemental analyses were performed on a Perkin-Elmer 2400 element analyser. TGA was analysed by using a Q50 thermogravimetric analyser. IR spectra were recorded on a Nicolet Impact 410 FTIR spectrometer. XPS measurements were performed on an ESCALAB 250 X-ray photoelectron spectroscopy, using Mg Kα X-ray as the excitation source. The 13 C NMR data were collected on a Bruker AVANCE IIIHD console with a 1.9-mm MAS probe. The scanning electron microscope analysis was performed on a JEOL JSM-6700F and Hitachi S-4800 field-emission scanning electron microscope (FE-SEM). ICP was performed on a Perkin-Elmer Elan DRC II Quadrupole Inductively Coupled Plasma Mass Spectrometer (ICP-MS) analyser. Synthesis of PAF-1-SH A re-sealable flask was charged with PAF-1 (200.0 mg), paraformaldehyde (1.0 g), glacial AcOH (6.0 ml), H 3 PO 4 (3.0 ml) and conc. HCl (20.0 ml). The flask was sealed and heated to 90 °C for 3 days. The resulting solid was collected, washed with water and methanol, and then dried under vacuum to produce yellow solid of PAF-1-CH 2 Cl. Subsequently the obtained PAF-1-CH 2 Cl was mixed with NaHS (1.2 g, 21.0 mmol) in 100 ml EtOH under N 2 and stirred at 75 °C for 3 days. The resulting solid was collected, washed with water and methanol, and then dried under vacuum to produce PAF-1-SH as yellow powder. Elemental Analysis: C: 72.5%; H: 4.24%; S: 17.6%. Synthesis of MCM-41-SH The MCM-41-SH was synthesized according to the procedures reported in the literature [14] . Elemental analysis: C: 8.54%; H: 1.81; S: 4.99%. Hg(II) sorption kinetics A 50 ml aqueous of Hg(NO 3 ) 2 (10 p.p.m., pH=6.8 NaH 2 PO 4 /Na 2 HPO 4 buffer) was added to an Erlenmeyer flask. Then 25.0 mg PAF-1-SH sample was added to form a slurry. The mixture was stirred at room temperature for 8 h. During the stirring period, the mixture was filtered at intervals through a 0.45-μm membrane filter for all samples, then the filtrates were analysed using ICP-MS to determine the remaining Hg(II) content. Hg(II) sorption isotherm PAF-1-SH (10.0 mg) was added to each Erlenmeyer flask containing Hg(NO 3 ) 2 solution (50 ml) with different concentrations. The mixtures were stirred at room temperature for 12 h, and then were filtered separately through a 0.45-μm membrane filter, and the filtrates were analysed by using ICP-MS to determine the remaining Hg(II) content. Ion selectivity tests Fifty milligrams of PAF-1-SH sample was added into an Erlenmeyer flask containing a 50-ml aqueous solution of Hg(NO 3 ) 2 , Pb(NO 3 ) 2 , NaAsO 2 , Cd(NO 3 ) 2 , Zn(NO 3 ) 2 , Ca(NO 3 ) 2 , Mg(NO 3 ) 2 with sorts of concentration in NaH 2 PO 4 /Na 2 HPO 4 buffer (pH=6.8). The mixture in the form of slurry was stirred at room temperature for 12 h, and then was filtered through a 0.45-μm membrane filter, and the filtrates were analysed using ICP-MS to determine the contents. Breakthrough experiments Hundred milligrams of PAF-1-SH sample was packed into a pipette to form an adsorption column with inner diameter of ~3.3 mm and the packed sample length was about 7.8 cm. An aqueous solution (30 ml) of Hg(NO 3 ) 2 , Pb(NO 3 ) 2 , NaAsO 2 , Cd(NO 3 ) 2 , Zn(NO 3 ) 2 , Ca(NO 3 ) 2 , Mg(NO 3 ) 2 with sorts of concentration in NaH 2 PO 4 /Na 2 HPO 4 buffer (pH=6.8) was then passed through the column, and the filtrates were analysed using ICP-MS to determine the contents. How to cite this article: Li, B. et al. Mercury nano-trap for effective and efficient removal of mercury(II) from aqueous solution. Nat. Commun. 5:5537 doi: 10.1038/ncomms6537 (2014).